Arginylation regulates purine nucleotide biosynthesis by enhancing the activity of phosphoribosyl pyrophosphate synthase Protein arginylation is an emerging post-translational modification that targets a number of metabolic enzymes; however, the mechanisms and downstream effects of this modification are unknown. Here we show that lack of arginylation renders cells vulnerable to purine nucleotide synthesis inhibitors and affects the related glycine and serine biosynthesis pathways. We show that the purine nucleotide biosynthesis enzyme PRPS2 is selectively arginylated, unlike its close homologue PRPS1, and that arginylation of PRPS2 directly facilitates its biological activity. Moreover, selective arginylation of PRPS2 but not PRPS1 is regulated through a coding sequence-dependent mechanism that combines elements of mRNA secondary structure with lysine residues encoded near the N-terminus of PRPS1. This mechanism promotes arginylation-specific degradation of PRPS1 and selective retention of arginylated PRPS2 in vivo . We therefore demonstrate that arginylation affects both the activity and stability of a major metabolic enzyme. tRNA-dependent post-translational addition of Arg to proteins (arginylation) is mediated by arginyltransferase ATE1 (ref. 1 ), an enzyme that is conserved in all eukaryotic species and has been recently proposed to carry global regulatory functions [2] , [3] , [4] . In higher eukaryotes, ATE1 is essential for viability and has been shown to target a variety of protein substrates and to affect the development and functioning of the cardiovascular system, cell migration and neural crest-dependent morphogenesis [2] , [3] , [4] , [5] , [6] , [7] . Recent studies from our lab identified over 100 proteins arginylated in vivo , including a prominent subset of metabolic enzymes, as well as proteins related to the actin cytoskeleton [3] , [7] , [8] . While the impact of arginylation on metabolism is still unclear, functional studies demonstrated its critical role in cell migration, which is dependent on N-terminal arginylation of β-actin [5] . β-Actin arginylation is selectively achieved via a coding sequence-dependent mechanism that relates its translation speed to arginylation-dependent ubiquitination and degradation and distinguishes it from the closely related γ-actin isoform, which is not normally arginylated in vivo [9] . This type of regulation sheds light on some of the underlying mechanisms that govern functional distinction between these two closely homologous actin isoforms, which do not display marked difference in their amino-acid sequence or tertiary structure but are encoded by separate genes and carry distinct biological functions. Notably, such phenomenon of differential arginylation of closely related protein isoforms is not limited to cytoskeletal proteins. Another pair of differentially arginylated protein isoforms identified in our previous proteomics screen includes phosphoribosyl pyrophosphate synthases 1 and 2 (PRPS1 and PRPS2) (ref. 3 ). These two proteins catalyse the adenosine triphosphate (ATP)-dependent conversion of ribose 5- phosphate to phosphoribosyl pyrophosphate with the help of ATP, producing adenosine monophosphate (AMP) and 5-phosphoribosyl-1-pyrophosphate. This reaction constitutes the first step of de novo purine biosynthesis, and is essential for normal metabolism [10] , [11] . Multiple studies suggest that PRPS isoforms play distinct roles in normal physiology and disease, but overall the underlying molecular mechanisms of functional distinction between PRPS isoforms are not fully understood. A recent study shows a specific role of PRPS2 in Myc-driven carcinogenesis and identifies PRPS2 as a specific protein factor that couples nucleotide biosynthesis and metabolic rate in cancer cells [12] . Notably, our prior data identifies a specific N-terminal arginylation site on Asn3 of PRPS2, which distinguishes it from the closely homologous PRPS1, which is not found to be arginylated on this site [3] . Such selective arginylation cannot be explained by the preferential recognition of PRPS2 by arginyltransferase, since the sequence context and structure in the vicinity of Asn3 is virtually identical between the two PRPS isoforms ( Supplementary Fig. 1 ). Similar to the case of β- and γ-actins, these two PRPS isoforms are encoded by different genes and are 96% identical at the amino-acid level; however, they only have 80% identity at the nucleotide level due to synonymous substitutions throughout the coding sequence ( Supplementary Fig. 1 ). The similarity of these two cases strongly invite testing whether the differential degradation effect of arginylation as observed by us in actin regulation also applies to these two closely homologous PRPS isoforms, and whether such a differentiation may contribute to an arginylation-dependent functional regulation. Here we studied the underlying mechanisms of differential arginylation of PRPS1 and PRPS2 and its downstream effects. We found that, like in the case of β- and γ-actins, these two PRPS isoforms are also distinguished by differential degradation after arginylation; however, this differentiation in the case of PRPS utilizes a broader mechanism that combines stable messenger RNA (mRNA) secondary structure elements and the presence/absence of Lys residues encoded in specific positions near the N-terminus of PRPS1 but not PRPS2. Moreover, we demonstrate that arginylation facilitates intracellular activity of PRPS2 and that lack of arginylation in cells leads to decreased robustness of purine nucleotide synthesis and increased rates of Ser/Gly biosynthesis. Our study constitutes the first demonstration of an enzyme’s intracellular activity being directly regulated by protein arginylation with consequences to cell metabolism, and suggests the existence of a general mechanism of coding sequence-dependent differential effect of arginylation on the metabolic stability of closely related protein isoforms, which involves a combination of Lys codons and structural features within the coding regions of their mRNA. Our study sheds the first light on the arginylation-dependent regulation of nucleotide biosynthesis and suggests a global role of arginylation in regulating metabolism in vivo . Ate1 knockout cells have impaired purine biosynthesis Our previous studies strongly suggest that arginylation constitutes a global process that likely regulates major physiological pathways. However, the effects of arginylation on cell metabolism were never reported. To address this question, we tested the overall effects of arginylation on cell sensitivity to treatment with different metabolic inhibitors. To do that, we compared viability of wild-type (WT) and arginylation-deficient Ate1 knockout (KO) mouse embryonic fibroblasts (MEFs) in the presence of different bioactive compounds from two chemical libraries (LOPAC1280 (Sigma) and Spectrum2000 (MicroSource Discovery Systems, Inc.)). Remarkably, out of the 3,280 compounds in these libraries, only 3 showed a profound selective toxicity towards Ate1 KO cells. These molecules include thioguanine, mercaptopurine and fluorouracil; all three are known antagonists of the nucleotide biosynthesis ( Fig. 1 , left column). To confirm the specificity of this effect to nucleotide metabolism, we tested whether the selective toxicity of these compounds towards Ate1 KO cells may be suppressed by the presence of added nucleoside and deoxyribonucleoside mixtures. We found that such an addition selectively abolishes the toxicity of thioguanine and mercaptopurine, the antagonists of purine nucleotide biosynthesis. No significant rescue effects were observed in the presence of fluorouracil, which acts on pyrimidine nucleotide biosynthesis ( Fig. 1 , bottom row). Thus, Ate1 KO cells appear to have selective impairments in the purine nucleotide biosynthesis pathway. 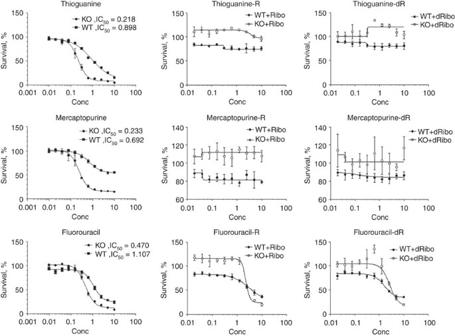Figure 1: Ate1 KO cells are sensitive to purine biosynthesis inhibitors. WT and Ate1 KO cell viability curves in the presence of increasing doses of nucleotide biosynthesis inhibitors alone (left) or in the presence of ribonucleosides (Ribo) and deoxyribonucleosides (dRibo) added to the tissue culture media. Error bars represent s.e.m. from four independent measurements. Figure 1: Ate1 KO cells are sensitive to purine biosynthesis inhibitors. WT and Ate1 KO cell viability curves in the presence of increasing doses of nucleotide biosynthesis inhibitors alone (left) or in the presence of ribonucleosides (Ribo) and deoxyribonucleosides (dRibo) added to the tissue culture media. Error bars represent s.e.m. from four independent measurements. Full size image Ate1 KO leads to increased Ser and Gly synthesis One of the metabolic effects of impairments in purine nucleotide biosynthesis should be manifested at the amino-acid level, in particular, the biosynthesis of Ser and Gly, which are involved in the folate cycle, coupled to the activity of thymidilate synthase and ultimately to DNA synthesis. As a feedback, downregulation of the purine nucleotide biosynthesis pathway should lead to an upregulation of Ser and Gly synthesis [13] , [14] . To test whether such upregulation is observed in Ate1 KO and to determine the overall effect of the Ate1 KO on the synthesis of key intracellular metabolites, we used U- 13 C-glucose to label WT and Ate1 KO-cultured fibroblasts and quantified the overall 13 C labelling of intracellular metabolites using gas chromatography–mass spectrometry (GC–MS [15] , [16] ). While labelling of most metabolites was overall unchanged or somewhat lowered in Ate1 KO ( Supplementary Fig. 2 ), 13 C labelling of Ser and Gly was 1.5–2-fold higher in Ate1 KO cells compared with WT ( Fig. 2 ), suggesting that in these cells Ser and Gly synthesis occurs at a much higher rate than in control, and/or this synthesis prevails over salvaging of these amino acids from the medium. 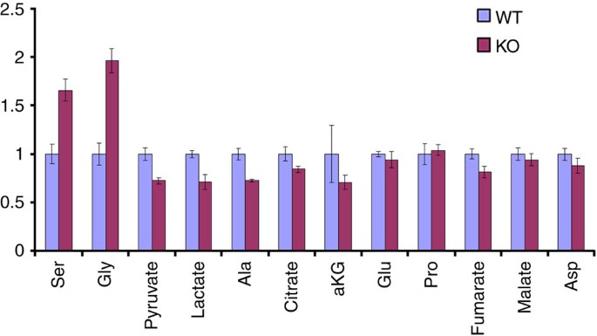Figure 2: Ate1 KO cells have increased Ser/Gly biosynthesis. Normalized13C labelling of intracellular metabolites in WT (blue bars) and Ate1 KO (red bars) cells. Error bars represent s.e.m. from two independent experiments analysed in triplicates. aKG: α-ketoglutarate. Figure 2: Ate1 KO cells have increased Ser/Gly biosynthesis. Normalized 13 C labelling of intracellular metabolites in WT (blue bars) and Ate1 KO (red bars) cells. Error bars represent s.e.m. from two independent experiments analysed in triplicates. aKG: α-ketoglutarate. Full size image Arginylation regulates intracellular activity of PRPS2 In search for potential protein targets that may underlie the increased sensitivity of Ate1 KO cells to the inhibitors of purine nucleotide biosynthesis, we turned to the results of our previous screens for proteins arginylated in vivo [17] , where two closely related enzymes of purine biosynthesis, PRPS1 and PRPS2, were found to be differentially arginylated at the N-terminus. These enzymes in principle affect both purine nucleotide and Ser/Gly biosynthesis, and thus represent good candidates for the metabolic changes observed in Ate1 KO cells. To test whether arginylation differentially regulates these enzymes, we first compared the overall amounts of endogenous PRPS in WT and Ate1 KO cells and found that Ate1 KO cells contained more total PRPS protein than WT cells ( Fig. 3a ). However, when we measured the activity of PRPS in the WT and Ate1 KO cells by measuring the specific generation of AMP from PRPS substrates ribose 5′-phosphate and ATP per unit of enzyme [18] , we found that PRPS in WT cells has a higher unit activity than in the Ate1 KO cells. Thus, arginylation in WT cells enhances the overall activity of PRPS ( Fig. 3b ). 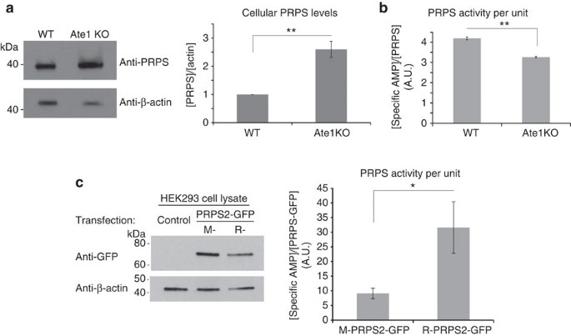Figure 3: The enzymatic activity of PRPS2 is increased by N-terminal arginylation. (a) Immunoblots of WT and Ate1 KO cell lysates probed with anti-PRPS and -β-actin as a loading control show that endogenous PRPS levels are higher in Ate1 KO cells compared with WT, opposite to the metabolic effects in these cells that suggest a reduction in PRPS function. (b) Total PRPS activity measured as AMP levels in WT and Ate1 KO cell extracts, normalized to PRPS levels shown ina. Ate1 KO cells have reduced total PRPS activity. (c) Normalized unit activity of non-arginylated (M-) and arginylated (R-) PRPS2 activity measured as AMP levels in soluble extracts from HEK293T cells transfected with non-arginylated or constitutively arginylated GFP-fused PRPS2 (M-PRPS2-GFP and R-PRPS2-GFP, respectively) (see alsoSupplementary Table 1). For each measurement, the levels of endogenous PRPS activity in untransfected cells was determined in the same experiment and subtracted from the total values, which were further normalized by the concentrations of the GFP-fused recombinant PRPS2 to reflect only the comparative unit activity of the expressed M- or R-PRPS2. Error bars represent s.e.m. (n=3). **P<0.01; *P<0.05. Figure 3: The enzymatic activity of PRPS2 is increased by N-terminal arginylation. ( a ) Immunoblots of WT and Ate1 KO cell lysates probed with anti-PRPS and -β-actin as a loading control show that endogenous PRPS levels are higher in Ate1 KO cells compared with WT, opposite to the metabolic effects in these cells that suggest a reduction in PRPS function. ( b ) Total PRPS activity measured as AMP levels in WT and Ate1 KO cell extracts, normalized to PRPS levels shown in a . Ate1 KO cells have reduced total PRPS activity. ( c ) Normalized unit activity of non-arginylated (M-) and arginylated (R-) PRPS2 activity measured as AMP levels in soluble extracts from HEK293T cells transfected with non-arginylated or constitutively arginylated GFP-fused PRPS2 (M-PRPS2-GFP and R-PRPS2-GFP, respectively) (see also Supplementary Table 1 ). For each measurement, the levels of endogenous PRPS activity in untransfected cells was determined in the same experiment and subtracted from the total values, which were further normalized by the concentrations of the GFP-fused recombinant PRPS2 to reflect only the comparative unit activity of the expressed M- or R-PRPS2. Error bars represent s.e.m. ( n =3). ** P <0.01; * P <0.05. Full size image To test whether the selective arginylation of PRPS2 facilitates its activity, we compared PRPS activity in cell extracts prepared from human embryonic kidney (HEK)293T cells transfected with either non-arginylated or constitutively arginylated PRPS2. To ensure that this measurement is restricted only to the transfected PRPS2, and not to the endogenous activity of PRPS enzyme, we performed a separate measurement of endogenous PRPS activity in untransfected cell extracts and subtracted it as the background. To exclude the effect of potentially altered protein levels between transfections on the activity readings, each measurement was normalized to the concentration of the transfected protein ( Table 1 ). Thus, the end measurement in these assays represented normalized activity of transfected PRPS2 above the endogenous background. Remarkably, these assays showed that AMP levels generated by arginylated PRPS2 per enzyme unit were nearly threefold higher than the non-arginylated one, suggesting that N-terminal arginylation greatly facilitates the enzymatic activity of PRPS2 ( Fig. 3b ). Table 1 AMP production as an indicator of the enzymatic activity of various forms of PRPS. Full size table Arginylated PRPS2 is selectively resistant to degradation Many cell types, including those used in our studies, contain two major PRPS isoforms, PRPS1 (which is generally more ubiquitous) and PRPS2 (which is more cell-type specific and more tightly regulated). These two proteins are highly similar in their amino-acid sequence, including their N-termini where PRPS2 is arginylated. We have previously found that such selective arginylation of closely related protein isoforms can be regulated through their differential degradation [9] . To test whether selective arginylation of PRPS2, but not the closely related PRPS1, may be regulated by such degradation-dependent mechanisms, we tested the metabolic stability of exogenously expressed constitutively arginylated and non-arginylated PRPS1 and 2 (M-PRPS1/2 and R-PRPS1/2, respectively), expressed in HEK293T cells as green fluorescent protein (GFP) fusions, using the ubiquitin fusion technique previously employed in our studies, which enables expression of proteins with different amino-acid residues at the N-terminus ( Fig. 4a ). This analysis revealed that, while both PRPS isoforms are at least partially destabilized upon arginylation, R-PRPS2 is much more metabolically stable than R-PRPS1 ( Fig. 4b ). This effect is co-translational since, once synthesized, both the arginylated and non-arginylated forms of PRPS isoforms remain relatively stable over time in the presence of cycloheximide that inhibits de novo protein synthesis (an assay that measures specifically the rate of post-translational but not co-translational degradation) [9] ( Fig. 5a,b ). Moreover, this effect is likely ubiquitin dependent since ubiquitination levels of PRPS1 (both M- and R-forms) are much higher than PRPS2 ( Fig. 5c ). Thus, selective arginylation of PRPS2 in vivo is likely achieved through specific ubiquitin-dependent degradation of R-PRPS1 but not R-PRPS2. 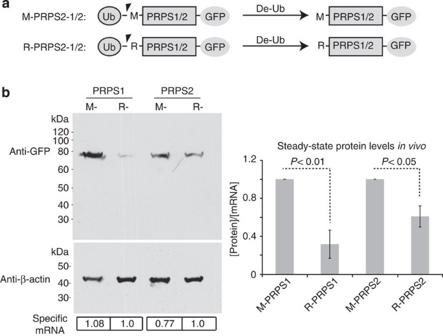Figure 4: N-terminal arginylation differentially affects protein stability of PRPS1 and PRPS2. (a) Linear maps of the recombinant constructs representing constitutively non-arginylated or arginylated forms of PRPS1/2. When expressedin vivo, the N-terminal ubiquitin moiety is removed during translation by de-ubiquitinating (De-Ub) enzymes, exposing the Met (M-) or Arg (R-) at the protein’s N-terminus (arrowheads). (b) Left: representative immunoblots of the steady-state levels of non-arginylated (M-) and constitutively arginylated (R-) recombinant PRPS expressed as GFP fusions in HEK293T cells. The concentration of specific mRNA in each sample was quantified by quantitative PCR using GFP-specific primers and actin primers as control and then normalized to the values of the R- samples separately for PRPS1 or PRPS2. Right: average steady-state levels of M- and R- PRPS1 and PRPS2 proteins per unit of specific mRNAin vivo. The value of R-PRPS1 was normalized to that of M-PRPS1. Similarly, R-PRPS2 was normalized to M-PRPS2. Error bars represent s.e.m. (PRPS1/2:n=4). Figure 4: N-terminal arginylation differentially affects protein stability of PRPS1 and PRPS2. ( a ) Linear maps of the recombinant constructs representing constitutively non-arginylated or arginylated forms of PRPS1/2. When expressed in vivo , the N-terminal ubiquitin moiety is removed during translation by de-ubiquitinating (De-Ub) enzymes, exposing the Met (M-) or Arg (R-) at the protein’s N-terminus (arrowheads). ( b ) Left: representative immunoblots of the steady-state levels of non-arginylated (M-) and constitutively arginylated (R-) recombinant PRPS expressed as GFP fusions in HEK293T cells. The concentration of specific mRNA in each sample was quantified by quantitative PCR using GFP-specific primers and actin primers as control and then normalized to the values of the R- samples separately for PRPS1 or PRPS2. Right: average steady-state levels of M- and R- PRPS1 and PRPS2 proteins per unit of specific mRNA in vivo . The value of R-PRPS1 was normalized to that of M-PRPS1. Similarly, R-PRPS2 was normalized to M-PRPS2. Error bars represent s.e.m. (PRPS1/2: n =4). 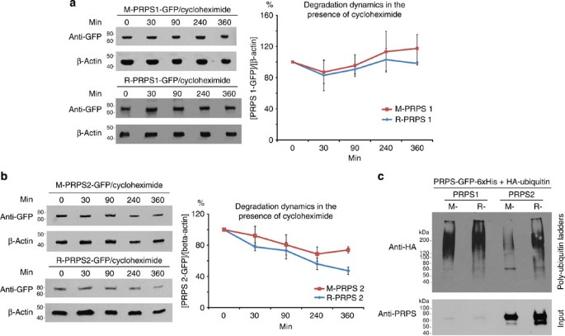Figure 5: Post-translational degradation curves and ubiquitination levels of PRPS enzymes. (a,b) Post-translational degradation of M- and R-PRPS1 and -PRPS2. In each set, the left panel shows a representative immunoblot and the right panel shows quantification of three independent repeats. Error bars represent s.e.m. The effectiveness of the cycloheximide treatment in these experiments was validated by measuring the degradation of the cyclin D1 on the same blot, as shown inSupplementary Fig. 3. (c) Ubiquitination levels of M- and R-PRPS1 and -PRPS2. Full size image Figure 5: Post-translational degradation curves and ubiquitination levels of PRPS enzymes. ( a , b ) Post-translational degradation of M- and R-PRPS1 and -PRPS2. In each set, the left panel shows a representative immunoblot and the right panel shows quantification of three independent repeats. Error bars represent s.e.m. The effectiveness of the cycloheximide treatment in these experiments was validated by measuring the degradation of the cyclin D1 on the same blot, as shown in Supplementary Fig. 3 . ( c ) Ubiquitination levels of M- and R-PRPS1 and -PRPS2. Full size image Our data demonstrate that the biological activity of a key metabolic enzyme can be facilitated by its arginylation, and suggest that selective regulation of PRPS2 by arginylation likely plays a key role in purine nucleotide biosynthesis by facilitating the activity of this enzyme in vivo . This finding thus expands the traditional views on the role of arginylation in regulating its target proteins. It has been previously shown that arginylation can facilitate protein turnover as a part of the ubiquitin-dependent N-end rule pathway, and that it can also regulate protein–protein interactions and facilitate their assembly and intracellular dynamics, as seen for actin at the cell leading edge [5] and talin fragment in cell–cell adhesion [19] . The current study expands the scope of biological functions of arginylation by demonstrating that this modification can also affect enzymatic activity and regulate nucleotide metabolism in vivo , placing this emerging post-translational modification in line with other major modifications that regulate activity of key enzymes in major metabolic pathways. We have previously shown that selective arginylation of closely homologous actin isoforms can constitute an underlying factor that ensures their functional distinction through a mechanism that couples differences in their nucleotide protein-coding sequence, rather than amino-acid sequence, resulting in selective degradation of arginylated γ-actin, and retention and functional regulation of arginylated β-actin [9] . Importantly, the majority of arginylation-mediated degradation appears to take place co-translationally, both in the case of actin isoforms [9] and in the currently reported case of PRPS. It is likely that in the case of PRPS this selective degradation of arginylated PRPS1 but not PRPS2 is mediated both by their nucleotide-coding sequence and by the presence of N-terminally positioned Lys residues, similarly to actin [9] . Detailed comparison of the amino-acid sequences and mRNA structures in the vicinity of the arginylated site, reveals two prominent differences that could potentially underlie the selective degradation of R-PRPS1. First, PRPS1 contains two Lys residues (Lys5 and Lys18, Fig. 6a ), which are absent in the homologous positions in PRPS2. Second, PRPS1 possesses notable differences in predicted mRNA structure in the 5′-region of its coding sequence when compared with PRPS2 ( Fig. 6b ). To test the contribution of these features to the stability of arginylated PRPS isoforms we performed mutagenesis studies and found that the effect of mutations in this area is opposite for the two PRPS isoforms. In R-PRPS1, mutation of K18 to Arg (R) increases its stability, while the K5R mutation has negligible effects. In R-PRPS2, introduction of K into position 5 but not into position 18 results in its destabilization ( Fig. 6c ). This apparent discrepancy is actually in good agreement with the predicted mRNA secondary structures in the vicinity of the arginylated sites ( Fig. 6b ). A stable hairpin structure (−14 kcal mole −1 ) in PRPS2 is located immediately downstream of codon 5, whereas the most stable RNA hairpin structure in PRPS1 (−17 kcal mole −1 ) is predicted immediately downstream codon 18 ( Fig. 6b ). In both cases free-energy values of local stable secondary structures are lower than the previously proposed threshold values that can shape gene expression levels and, specifically, to obstruct translation [20] . Thus, these predicted RNA stable hairpins would be expected to lead to ribosome pausing at position 5 during translation of PRPS2 and at position 18 during translation of PRPS1, leading to differential effects of Lys in these positions and on the stability of protein translated from these two transcripts. While codon optimization may also affect translation speeds, we did not find any substantial difference between PRPS1 and PRPS2 that could explain the differential effect of K5, although a pair of rare codons near position 28 in PRPS1 may potentially contribute to the degradation effect of K18. Overall, the results of the current study, as well as the previously published study on the actin isoforms [9] , suggest that differential arginylation may constitute a general, previously unknown, mechanism of post-translational regulation of closely homologous proteins [21] . Identifying other proteins that undergo such regulation, and possibly the involvement of other post-translational modifications in similarly regulated processes, constitutes an exciting direction of future studies. 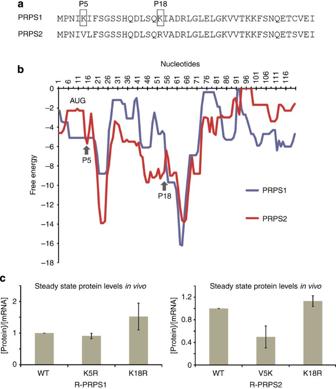Figure 6: Stability of arginylated PRPS depends on mRNA structure and the N-terminally encoded Lys. (a) Comparison of the amino-acid sequences of the N-terminal regions of PRPS1 and PRSP2. Boxes show the locations of important positions (5 and 18) for lysine residues that only exist in PRPS1 but not in PRPS2. (b) The free-energy profiles of mRNA folding along the nucleotide sequences of PRPS1 and PRPS2 transcripts in the vicinity of start codons predicted using window lengths of 30 nt. The positions of the start codon AUG, as well as codon positions 5 and 18 are indicated. (c) Left: steady-state levels of R-PRPS1 expressed as a native sequence (WT) or with point mutations at ubiquitination-eligible Lys residues to Arg (K5R and K18R). Error bars represent s.e.m. (n=3). Right: steady-state levels of native R-PRPS2 (WT) or with point mutations at positions 5 and 18 to ubiquitination-eligible Lys (V15K and R18K). Error bars represent s.e.m. (n=3). Figure 6: Stability of arginylated PRPS depends on mRNA structure and the N-terminally encoded Lys. ( a ) Comparison of the amino-acid sequences of the N-terminal regions of PRPS1 and PRSP2. Boxes show the locations of important positions (5 and 18) for lysine residues that only exist in PRPS1 but not in PRPS2. ( b ) The free-energy profiles of mRNA folding along the nucleotide sequences of PRPS1 and PRPS2 transcripts in the vicinity of start codons predicted using window lengths of 30 nt. The positions of the start codon AUG, as well as codon positions 5 and 18 are indicated. ( c ) Left: steady-state levels of R-PRPS1 expressed as a native sequence (WT) or with point mutations at ubiquitination-eligible Lys residues to Arg (K5R and K18R). Error bars represent s.e.m. ( n =3). Right: steady-state levels of native R-PRPS2 (WT) or with point mutations at positions 5 and 18 to ubiquitination-eligible Lys (V15K and R18K). Error bars represent s.e.m. ( n =3). Full size image While both PRPS1 and PRPS2 are commonly expressed in multiple cell types, it has been recently found that PRPS2, unlike PRPS1, possesses additional translational regulatory elements that enable it to function as a master regulator coupling protein and nucleotide biosynthesis and driving the elevated metabolic rate during Myc-driven tumorigenesis [12] . Our data that PRPS2, in contrast to PRPS1, is regulated by arginylation demonstrates an additional molecular switch that can specifically target PRPS2 activity. It appears likely that this selectivity reflects the additional importance of PRPS2 and could pose means of its tighter regulation during the coordination of nucleotide biosynthesis, translation and cancer. Unravelling the pathways involved in this regulation constitutes an exciting direction of further studies. Molecular cloning PRPS1 and PRPS2 were cloned from complementary DNA library prepared from MEFs using the following primers: Forward primer for M-PRPS1: 5′-ATG CCC GCG GTG GTA TGC CGA ATA TCA AAA TCT TCA GCG GGA-3′ Forward primer for R-PRPS1: 5′-ATC GCC GCG GTG GTA GGA ATA TCA AAA TCT TCA GCG GGA GCT CCC AC-3′ Forward primer for M-PRPS2: 5′-ATG CCC GCG GTG GTA TGC CTA ACA TCG TGC TCT TCA GCG G-3′ Forward primer for R-PRPS2: 5′-ATC GCC GCG GTG GTA GGA ACA TCG TGC TCT TCA GCG GCA GT-3′ Reverse primer for PRPS2: 5′-ATG CGG ATC CCC AGT GGG ACA TGG CTG AAC AGA TAG GAC A-3′ No mutations were found in the cloned sequences by validation with published sequences in public-accessible National Center for Biotechnology Information database. The third isoform of PRPS (PRPS3) is specifically expressed in testis but not in fibroblasts. Therefore it was not included in this study. The construction of constitutively arginylated or non-arginylated forms of PRPS1 and PRPS2 was performed using the Ub fusion technique, by insertion of an N-terminal Ub moiety upstream of the first codon of PRPS [9] . C-terminal GFP fusion was used to facilitate the detection of these recombinant proteins. Cell culture HEK293T cells (clone #T7) were purchased from ATCC. MEFs were isolated from littermate WT and Ate1 KO E12.5 mouse embryos and immortalized spontaneously by continuous passaging in culture [5] . All cells were maintained in equal mixture of DMEM medium (high glucose with Glutamax, Life Technologies) and F10 nutrient mix (Life Technologies) supplemented with 10% fetal bovine serum (Sigma) and antibiotics at 37 o C with 5% CO 2 . Cell transfection and expression of recombinant proteins Cells were split by using brief trypsin treatment 1 day before the experiment and allowed to grow to ∼ 75% confluency. Cells were transfected using Lipofectamine reagent (Life Technologies) according to the manufacturer’s protocol. To avoid the formation of protein aggregates due to overexpression, cells were incubated for <16 h after the initiation of the transfection. Lack of fluorescent aggregates in cells was confirmed by fluorescence microscopy. Western blots Cells were collected by scraping and washed briefly in PBS. After complete removal of supernatant, the cell pellets were weighed and then resuspended in 10 × w-v of 1 × SDS loading buffer, loaded onto SDS–PAGE and transferred to nitrocellulose membranes. GFP-fused protein was probed with mouse anti-GFP antibody (1:1,000, Roche, catalogue # 11814460001). Total PRPS proteins was probed with mouse anti-PRPS1/2/3 (1:1,000, Santa Cruz Biotech, sc-376440). Endogenous actin was probed with anti-actin (1:2,000, Cytoskeleton Inc., catalogue # AAN01) or monoclonal anti-β-actin (1:20,000, Sigma Aldrich, catalogue # A5441, clone AC-1). Visualization of the protein bands was performed with the secondary antibodies and reagents provided in the BM Chemifluorescence Western Blotting Kit Mouse/Rabbit (Roche) or the SuperSignal West Femto Chemiluminescence Kit (Pierce). Secondary antibodies from both kits were used at 1:5,000 dilution. Multiple exposures of X-ray films were taken to ensure only the signals within the linear range were to be used for analysis. Documentation and quantification of the results were performed according to our published protocol [9] , by scanning the X-ray films using an Epson 4490 Perfection scanner into grey scale digital files with 1,200 d.p.i. and analysing the density of the protein bands using ImageQuantTL (version7.0, GE Health Care), with the background being subtracted using built-in function of the analysis software. mRNA quantification Total RNA in cell samples was purified by RNeasy kit (Qiagen) followed by reverse transcription PCR and quantitative PCR analyses using GFP-specific primers (5′-TCAAGGACGACGGCAACTAC-3′ and 5′-TTGTGCCCCAGGATGTTGCC-3′) and human GAPDH-specific primers as a control (5′-CCAGGTGGTCTCCTCTGACTTC-3′ and 5′-GTGGTCGTTGAGGGCAATG-3′). Most mRNA samples were analysed in triplicates. mRNA secondary structure and codon optimization analysis mRNA secondary structure predictions were performed similarly to the analysis of actin isoforms [9] , using Afold program [22] and the RNA Mfold software [23] . Energy minimization was performed by a dynamic programming method that employs nearest neighbour parameters to evaluate free energy and finds the secondary structures with the minimum free energy by summing up the contributions from stacking, loop length and other structural features, using improved thermodynamic parameters [24] . Results were presented as the free-energy profiles of mRNA folding along the nucleotide sequences of interest with 30-nt window lengths, considering that about 30 nt of the mRNA are wrapped around the small ribosome subunit during translation. The local minima of free-energy profiles in the vicinity of start codons were estimated by taking into account the characteristic features (location of specific amino acids and frame length) of analysed transcripts. The analysis of codon optimization was performed using Graphical Codon Usage Analyzer 2.0 ( http://gcua.schoedl.de ) by comparing with the mouse ( Mus musculus ) relative codon usage table. Metabolic labelling of cells and analysis of the metabolites Cells were labelled and analysed using the procedure described in ref. 15 , as follows. For labelling, cultured WT and ATE1 KO cells were incubated for 8 h in MEM medium containing 2 g l −1 (50% U- 13 C-) glucose, 2 mM L -glutamine, 10% fetal bovine serum and 1 × non-essential amino-acid supplement. Following the labelling, cells were collected by scraping and centrifugation and resuspended in 0.6 ml cold (−20 °C) 50% methanol (in water) containing 100 μM L -norvaline (internal standard). The suspension was incubated on dry ice for 30 min, then thawed on ice for 10 min and centrifuged. The liquid phase was removed to a separate tube and 0.3 ml chloroform was added to the pellet. The tube was vortexed (5 × 15 s) before centrifuging for 5 min at 14,000 g at 4 °C. The top (methanol extract) layer was dried by centrifugal evaporation and stored at −80 o C before analysis. For the analysis, dried methanol extracts were derivatized first by addition of 50 μl 20 mg ml −1 of ethylhydroxylamine (Sigma, in dry pyridine) and incubation for 20 min at 80 °C. After cooling, 50 μl N -tert-butyldimethylsilyl- N -methyltrifluoroacetamide (Sigma) was added and samples were re-incubated for 60 min at 80 °C before centrifuging for 5 min at 14,000 g at 4 °C. The supernatant was transferred to an autosampler vial for GC–MS analysis. A Shimadzu QP2010 Plus GC–MS was programmed with an injection temperature of 250 °C, injection split ratio 1/10, with (typically) injection volume 0.5 μl. GC oven temperature started at 110 °C for 4 min, rising to 230 °C at 6 °C min −1 and to 280 °C at 20 °C min −1 with a final hold at this temperature for 2 min. GC flow rate with helium carrier gas was 50 cm s −1 . The GC column used was a 15 m × 0.25 mm × 0.25 μm SHRXI-5ms (Shimadzu). GC–MS interface temperature was 300 °C and (electron impact) ion source temperature was 200 °C, with 70 V/150 μA ionization voltage/current. The mass spectrometer was set to scan m/z range 50–600, with ∼ 1 kV detector sensitivity (modified as necessary). Metabolites were quantified using Metaquant [25] , with standard curves constructed using data from running varied amounts of mixtures of standards in the same batches as samples. Measurement of the activity of PRPS The methods were adapted from published protocols [18] . For MEFs, to minimize any potential effects from difference of cell growth, the WT and Ate1 KO cells were inoculated at low seeding density (<12.5% confluent in seeding) and grown to <50% confluent before collecting. For HEK293T cells, to minimize any potential effects from overexpression toxicity and/or protein aggregation, transfections were performed at 75% confluency and cells were collected within 14 h after transfection. Transfected or untransfected cells were scraped off culture dishes and washed briefly with PBS. The cell pellets were weighed and resuspended in 10 × volume of buffer A (2 mM N 2 HPO 4 , pH 7.4, 1 mM dithiothreitol and 1 mM EDTA) and cells were lysed by brief sonication on ice. The cell lysates were clarified by centrifugation at 40,000 g for 40 min at 4 o C in a Beckman Optima Max XP ultracentrifuge. The supernatants were then passed through a Sephadex G-25 column equilibrated with buffer A to remove small molecules (including endogenous nucleotides). The protein levels in the collected flow-through fractions were measured by the Bradford assay (Bio-Rad) and adjusted to equal concentration with buffer A. The final concentration of the cell extracts were in the range of 0.4 ∼ 0.8 mg ml −1 . For the transfected or non-transfected HEK293T cells, the level of PRPS–GFP in cell extracts was measured with anti-GFP in western blot (see Fig. 3c ). For MEFs, to increase the accuracy of comparison of enzyme activity between the WT and Ate1 KO cells, the cell extract from Ate1 KO was further diluted twofold. The levels of endogenous PRPS in all cell extracts were then measured with anti-PRPS in western blot (see Supplementary Fig. 4 ). Cell extracts were mixed with equal volume of reaction buffer (50 mM Tris–HCl, pH 7.4, 5 mM MgCl 2 , 1 mM EDTA, 1 mM dithiothreitol, 32 mM Na 3 PO 4 , 0.5 mM ATP, 0.15 mM ribose 5′-phosphate and 0.25 mM P 1 P 5 -diadenosine pentaphosphate Ap 5 A) at 37 °C for 15 min. To exclude the influence of any enzyme other than PRPS, reaction controls were set up for each sample, in which the PRPS-specific reaction substrate ribose 5′-phosphate was omitted from the buffer. At the end of the reaction, equal volume of 0.1 M EDTA was used to terminate the reaction. The reaction mixture is then filtered through Amicon cones with 30-kDa cutoff to collect the small molecule fraction for analysis. The HPLC-based end-point assay [26] was used for the measurement of AMP concentration in the reaction mixture, analysed in triplicates. The filtrates were injected into HPLC with ion-paired analytical Supelco C18 column (3 μm, 4.6 × 150 mm), and eluted at room temperature with 0.2 mM KH 2 PO 4 (pH 6) at a flow rate of 1.3 ml min −1 . Absorbance was measured at 254 nm. Standard curve for AMP was measured in the linear range of 5–17 μM. The samples were diluted two times in the running buffer before HPLC injection. The intensity of AMP peak was used to calculate AMP concentration from the standard curve and to evaluate the total activity of the enzyme. The amount of PRPS proteins in the cell extracts, as determined by western blot, was then used to normalize the enzyme activity per protein unit. Measurement of PRPS post-translational degradation Ate1 KO MEF stably transfected with the constitutive non-arginylated (M-) and arginylated (R-) forms of PRPS1 or PRPS2 were used in this experiment. To create agents for stable transfection, retroviruses carrying constitutive non-arginylated or arginylated PRPS1 or PRPS2 with a C-terminal GFP were constructed by transfecting HEK293T cells with the low-expression pBabe-Puro vectors carrying coding sequence for the desired proteins and the vectors of GAG-Pol and VSV-G vector [19] . The viruses were then allowed to infect Ate1 KO MEF in the presence of 10 mg ml −1 polybrene over the course of 3 days. Successfully transfected MEFs were enriched by drug selection with puromycin and then further enriched by fluorescence sorting. To inhibit de novo protein translation, cycloheximide was added to the culture medium of stably transfected MEFs to the concentration of 100 μg ml −1 . Cells were then collected in a series of time points for western blot analysis. To confirm the effects of the cycloheximide on protein degradation, cyclin D1, a protein with a known short half-life was used as internal control ( Supplementary Fig. 3 ). Measurement of ubiquitination of PRPS PRPS–GFP fusion proteins were conjugated with a C-terminal 6xHis tag for this experiment. HEK293T cells were co-transfected with the vector carrying desired PRPS constructs and a vector carrying N-terminal HA-tagged ubiquitin [9] . At 12 h post transfection, 20 μM of MG132 was added to culture media, followed by incubation for 6 h to allow for accumulation of ubiquitinated proteins. The transfected cells were then lysed with 8 M urea/PBS, pH 8.0 and PRPS were pulled down using NTA-Ni resin and washed several times with alternating buffers containing 8 M urea/PBS at pH 8.0 and pH 5.6. The polyubiquitin chains on the purified PRPS were then visualized using western blots with anti-HA antibody. Image processing Photoshop (from Adobe) was used to adjust the contract and brightness of representative images by linear adjustment of display levels applied to the whole image uniformly. Statistics Calculation of s.d. and s.e.m. was performed based on Student’s t -distribution. How to cite this article: Zhang, F. et al . Arginylation regulates purine nucleotide biosynthesis by enhancing the activity of phosphoribosyl pyrophosphate synthase. Nat. Commun. 6:7517 doi: 10.1038/ncomms8517 (2015).